Inhibition of Ebola virus glycoprotein-mediated cytotoxicity by targeting its transmembrane domain and cholesterol The high pathogenicity of the Ebola virus reflects multiple concurrent processes on infection. Among other important determinants, Ebola fusogenic glycoprotein (GP) has been associated with the detachment of infected cells and eventually leads to vascular leakage and haemorrhagic fever. Here we report that the membrane-anchored GP is sufficient to induce the detachment of adherent cells. The results show that the detachment induced through either full-length GP 1,2 or the subunit GP 2 depends on cholesterol and the structure of the transmembrane domain. These data reveal a novel molecular mechanism in which GP regulates Ebola virus assembly and suggest that cholesterol-reducing agents could be useful as therapeutics to counteract GP-mediated cell detachment. The current Ebola virus outbreak is the largest and most severe in the history of this virus. Ebola virus poses a threat to thousands of people in West Africa, with outbreaks reported in Guinea, Liberia, Sierra Leone and Nigeria [1] , [2] . Despite the devastating consequences of Ebola virus infection, the treatment options remain limited and experimental. Recently, the use of cholesterol-reducing agents as an adjuvant therapy to reduce the sepsis-like side effects of Ebola virus disease has been suggested [3] , [4] . The dysregulation of the immune response and a heavy inflammatory reaction, described as a ‘cytokine storm’, are induced on EBOV infection [5] . Whether the detachment of infected endothelial cells and the concomitant leakage of the endothelial barrier are important factors in the pathogenesis of Ebola virus disease remains controversial [6] , [7] , [8] , [9] , [10] , [11] . Among other factors, the cytotoxicity of EBOV has been attributed to the envelope glycoprotein (GP) [6] ; however, the molecular mechanism underlying the pathogenicity of this virus is unclear. GP is an essential virulence factor that plays a key role in viral entry, membrane fusion, epitope shielding and EBOV assembly [12] , [13] , [14] , [15] , [16] , [17] . Virulence has been attributed not only to the membrane-anchored GP but also to the soluble form of this protein, sGP, which results from RNA editing [18] . sGP increases endothelial permeability by acting as an activator of neutrophils and macrophages, which regulates the host immune response [19] , [20] , [21] , [22] . Recently, GP shedding was shown to impact endothelial permeabilization [23] . In addition, the interaction between β1-integrin and GP was shown to contribute to the loss of adhesion of GP-expressing cells [7] , [24] . Furthermore, a role for the GP 2 subunit in counteracting interferon-induced antiviral response via the protein tetherin (BST-2) has been proposed [25] . GP is a type I membrane protein that exhibits high N - and O -glycosylation, and undergoes proteolytical cleavage through furin in the trans -Golgi network, which yields the large amino-terminal GP 1 subunit and the small carboxy-terminal GP 2 subunit [26] . The GP 2 subunit contains a putative fusion peptide and a transmembrane domain (TMD) and is palmitoylated twice on the short cytoplasmic tail [27] , [28] . Owing to an intramolecular disulfide bond, GP 1 and GP 2 do not dissociate on furin cleavage [29] . The mature GP forms a trimer that comprises of disulfide-bridged GP 1,2 subunits [30] , [31] . The ectopic expression of GP is sufficient to induce the detachment of adherent cells [32] , and a mucin-like domain within subunit GP 1 has been suggested to strongly impact this process [6] . Cell detachment accounts for the loss of the endothelial barrier of infected blood vessels, which putatively leads to vascular leakage and contributes to the high pathogenicity of the virus [6] , [9] . Ebola virions are filamentous in shape, and the matrix protein VP40 and GP are sufficient to produce protrusions at the plasma membrane of adherent cells [33] , [34] . The protrusions resulting from VP40 are virus like, whereas the structures resulting from GP alone appear pleiomorphic [35] , [36] . The combination of VP40 and GP is sufficient to produce filamentous virus-like particles that exhibit the morphology of Ebola virions [37] , [38] . Here we report that GP-induced cell detachment might be attributed to the GP 2 subunit and that cytotoxicity is strongly impacted through cholesterol and a GXXXA motif in the TMD. Furthermore, we show that the GP 2 subunit induces filamentous protrusions at the plasma membrane that also depend on cholesterol and the GXXXA motif, which implies a role for GP in the assembly of the filamentous Ebola virus. A mucin-like domain within GP has been attributed to the induction of cell detachment [6] . The isolated GP 2 subunit has not been analysed in this context, and notably, the contribution of GP 2 to cell detachment or the production of virus-like filaments was not observed using yellow fluorescent protein (YFP)-GP 2 fusions [25] . These results left a possibility that the mucin-like domain, rather than being involved in mediating detachment, acts as a spacer to maintain an appropriate distance between GP 1 and GP 2 and thereby allow the interaction of GP 2 subunits ( Fig. 1a ). In this case, the deletion of the mucin-like domain then would reduce the relative distance of GP 1 to the membrane, causing GP 1 to interfere with the oligomerization of GP 2 . Accordingly, YFP-GP 2 might not induce cell detachment, as the bulky YFP moiety may have taken the role of GP 1 in the GP 1,2 -Δmucin construct, potentially disturbing GP 2 oligomerization and masking the contribution of this protein to cell detachment. 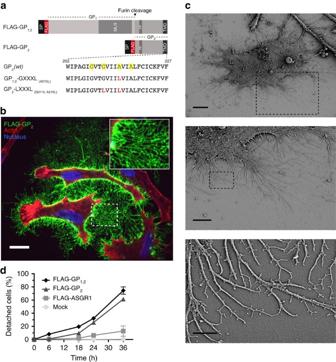Figure 1: The GP2subunit of Ebola GP leads to filament formation at the plasma membrane of HeLa cells and their detachment. (a) Constructs. All constructs are based on ZEBOV GP. For GP1,2constructs, a linker-flanked FLAG tag was positioned between the signal sequence and the GP1subunit. For GP2, the signal sequence of GP was fused to a linker-flanked FLAG tag, followed directly by GP2. GP variants are abbreviated as GP2-LXXXL (=FLAG-GP2-G211LA215L), and GP1,2-GXXXL (=FLAG-GP1,2-A215L). The respective domains are drawn to scale. SP, signal peptide; FLAG (epitope); MLR, mucin-like region; FP, fusion peptide. Gly and Ala residues seaming the TMD are highlighted (yellow boxes). (b) Immunofluorescence analysis of a HeLa cell transiently transfected with FLAG-GP2. Green, FLAG-GP2; red, actin; blue, nucleus. Scale bar, 10 μm. (c) Scanning electron microscopy of HeLa cells transiently transfected with FLAG-GP2at different magnifications. Dashed lines (inb,c): areas of inset. Scale bars indicate 10 μm (top), 5 μm (middle) and 1 μm (bottom). (d) Detachment of HeLa cells transiently transfected with either FLAG-GP1,2, -GP2, -ASGR1 (as a control) or mock-transfected cells within 36 h. Data points represent the mean±s.d. of three independent experiments (N=3). The ratio of adherent to detached cells was determined by flow cytometry. Black diamonds, GP1,2-transfected cells; light black triangles, GP2-transfected cells; dark grey squares, ASGR1-transfected cells; light grey circles, mock-transfected cells. Figure 1: The GP 2 subunit of Ebola GP leads to filament formation at the plasma membrane of HeLa cells and their detachment. ( a ) Constructs. All constructs are based on ZEBOV GP. For GP 1,2 constructs, a linker-flanked FLAG tag was positioned between the signal sequence and the GP 1 subunit. For GP 2 , the signal sequence of GP was fused to a linker-flanked FLAG tag, followed directly by GP 2 . GP variants are abbreviated as GP 2 -LXXXL (=FLAG-GP 2 -G211LA215L), and GP 1,2 -GXXXL (=FLAG-GP 1,2 -A215L). The respective domains are drawn to scale. SP, signal peptide; FLAG (epitope); MLR, mucin-like region; FP, fusion peptide. Gly and Ala residues seaming the TMD are highlighted (yellow boxes). ( b ) Immunofluorescence analysis of a HeLa cell transiently transfected with FLAG-GP 2 . Green, FLAG-GP 2 ; red, actin; blue, nucleus. Scale bar, 10 μm. ( c ) Scanning electron microscopy of HeLa cells transiently transfected with FLAG-GP 2 at different magnifications. Dashed lines (in b , c ): areas of inset. Scale bars indicate 10 μm (top), 5 μm (middle) and 1 μm (bottom). ( d ) Detachment of HeLa cells transiently transfected with either FLAG-GP 1,2 , -GP 2 , -ASGR1 (as a control) or mock-transfected cells within 36 h. Data points represent the mean±s.d. of three independent experiments ( N =3). The ratio of adherent to detached cells was determined by flow cytometry. Black diamonds, GP 1,2 -transfected cells; light black triangles, GP 2 -transfected cells; dark grey squares, ASGR1-transfected cells; light grey circles, mock-transfected cells. Full size image FLAG-GP2 induces protrusions at the plasma membrane We observed the presence of a seam-like arrangement of Gly and Ala residues with a central G/A/S-XXX-G/A/S motif in the TMD of GP 2 . These motifs are well-established hubs for TMD–TMD interactions [39] ; thus, these motifs likely contribute to the oligomerization of GP. To challenge the hypothesis that TMD–TMD interactions might be disrupted due to the steric hindrance resulting from the presence of a bulky protein (unduly close GP 1 in the mucin-like domain deletions or YFP in YFP-GP 2 ), we designed constructs based on the GP from Ebola Zaire (ZEBOV) by using a small FLAG tag directly fused to the GP 2 domain (as depicted in Fig. 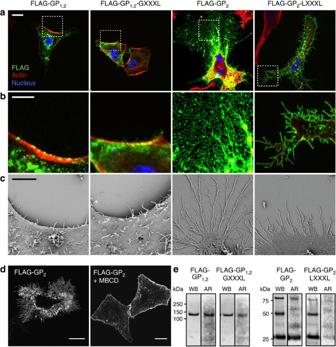Figure 2: The TMD of GP2affects the morphology of GP2-induced filaments. (a) HeLa cells were transiently transfected with FLAG-GP1,2, -GP1,2-GXXXL, -GP2or -GP2-LXXXL for 24 h. The cells were fixed, and FLAG-tagged proteins were visualized by immunofluorescence. Green, α-FLAG; red, actin; blue, nucleus. Dashed lines, area of inset. Scale bar, 10 μm. (b) Magnifications of the areas indicated ina. Scale bar, 5 μm. (c) Scanning electron microscopy images of cells transfected with the indicated constructs. Scale bar, 5 μm. (d) MBCD abolishes GP2-induced filaments at the plasma membrane. Immunofluorescence analysis of HeLa cells transiently transfected with FLAG-GP2for 24 h, and incubated with a final concentration of 0.5 mM MBCD 6 h post transfection. Scale bar, 20 μm. (e) GP variants exhibit differences in their ability to bind cholesterol. Photoaffinity labelling of full-length FLAG-GP1,2, -GP1,2-GXXXL, -GP2or -GP2-LXXXL using tritiated, photolabile cholesterol. HeLa cells were transiently transfected with the indicated constructs for 24 h. After 16 h, tritiated photocholesterol was added. The cells were then ultraviolet irradiated, lysed, subjected to immunoprecipitation against the FLAG epitope and analysed by western blot and digital autoradiography (Supplementary Fig. 8). AR, autoradiography; WB, western blot. 1a ; Supplementary Table 2 ). This tag, which contained eight amino acids (with a mass of ∼ 2 kDa, including the linker peptide), was not expected to exert strong steric hindrance. Surprisingly, immunofluorescence and scanning electron microscopy revealed that the transient transfection of HeLa and various other cell lines ( Supplementary Fig. 1 ) with FLAG-GP 2 constructs resulted in the drastic formation of filaments at the plasma membrane ( Fig. 1b,c and Fig. 2 ). The transfection of FLAG-GP 1,2 led to the formation of dot-like structures ( Fig. 2a,b , left panel) that likely resemble the previously described GP 1,2 -induced pleiomorphic structures [36] . The FLAG-GP 2 -induced filaments were, on average, 14.7±0.44 μm in length, and ∼ 50 nm in diameter ( Supplementary Fig. 3a ). The observed filament length is consistent with the dimensions observed for the virus-like particles produced through VP40 and GP 1,2 (ref. 36 ). The observed reduction in diameter (80 nm for virions) might reflect the lack of other viral proteins. The filaments exhibited a high extent of peripheral branching, with fine and widespread extensions ( Fig. 1b,c ). Strikingly, a strong reduction in the volume of the cells was observed concomitant with the production of these filaments and frequently resulted in rod-like cell remnants ( Fig. 1b ; Supplementary Movies 1–3 ). Figure 2: The TMD of GP 2 affects the morphology of GP 2 -induced filaments. ( a ) HeLa cells were transiently transfected with FLAG-GP 1,2 , -GP 1,2 -GXXXL, -GP 2 or -GP 2 -LXXXL for 24 h. The cells were fixed, and FLAG-tagged proteins were visualized by immunofluorescence. Green, α-FLAG; red, actin; blue, nucleus. Dashed lines, area of inset. Scale bar, 10 μm. ( b ) Magnifications of the areas indicated in a . Scale bar, 5 μm. ( c ) Scanning electron microscopy images of cells transfected with the indicated constructs. Scale bar, 5 μm. ( d ) MBCD abolishes GP 2 -induced filaments at the plasma membrane. Immunofluorescence analysis of HeLa cells transiently transfected with FLAG-GP 2 for 24 h, and incubated with a final concentration of 0.5 mM MBCD 6 h post transfection. Scale bar, 20 μm. ( e ) GP variants exhibit differences in their ability to bind cholesterol. Photoaffinity labelling of full-length FLAG-GP 1,2 , -GP 1,2 -GXXXL, -GP 2 or -GP 2 -LXXXL using tritiated, photolabile cholesterol. HeLa cells were transiently transfected with the indicated constructs for 24 h. After 16 h, tritiated photocholesterol was added. The cells were then ultraviolet irradiated, lysed, subjected to immunoprecipitation against the FLAG epitope and analysed by western blot and digital autoradiography ( Supplementary Fig. 8 ). AR, autoradiography; WB, western blot. Full size image Cytotoxicity of GP is encoded in its GP 2 subunit Next, we analysed the potential induction of HeLa cell detachment through FLAG-GP 2 . Although HEK cells are frequently used to study GP-induced detachment [6] , [32] , we performed quantitative measurements in HeLa cells, which adhere more strongly and are less prone to detachment than HEK cells. HeLa cells were transfected with either FLAG-GP 2 or FLAG-GP 1,2 constructs for various times, and the ratio of detached to adherent cells was determined through flow cytometry ( Fig. 1d ). As a control, we employed plasma membrane-resident ( Supplementary Fig. 3f ) asialoglycoprotein receptor 1 (ASGR1), which forms trimers similar to Ebola GP. At 36 h post transfection, ∼ 60% of the FLAG-GP 2 -transfected cells were detached, whereas ASGR1-transfected cells did not exceed 10% detachment, although the protein levels were higher ( Fig. 1d ). Importantly, FLAG-GP 1,2 -transfected cells achieved a similar degree of detachment ( ∼ 70%, after 36 h), which indicated that the propensity to induce detachment is attributed to the GP 2 subunit and not the mucin-like domain within GP 1 as previously reported [6] . A GXXXA motif in the TMD of GP impacts cytotoxicity Single G/A/S-XXX-G/A/S motifs are able to mediate TMD–TMD interactions [39] . We therefore speculated that the presence of multiple repeats of these motifs, aligned on one side of the TMD of GP ( Supplementary Fig. 5b ), would enhance GP oligomerization and potentially influence the extent of filament formation and detachment. To this end, we changed the central GXXXA motif in FLAG-GP 2 to LXXXL (as highlighted in Fig. 1a and Supplementary Fig. 5b ). This mutant was analysed through immunofluorescence and scanning electron microscopy. Notably, filament formation was strongly inhibited, with the average lengths reduced to 4.7±0.33 μm ( Supplementary Fig. 3a ). When the propensity of the mutant to confer detachment was analysed, a significant ∼ 50% reduction was observed compared with wild-type FLAG-GP 2 ( Fig. 3b ), which suggested that the GXXXA motif contributes to the extent of filament formation and GP 2 -mediated cell detachment. Strikingly, a single point mutation in full-length FLAG-GP 1,2 , yielding GP 1,2 -GXXXL, exhibited a drastic reduction of >50% in detachment compared with the wild-type construct ( Fig. 3a ). 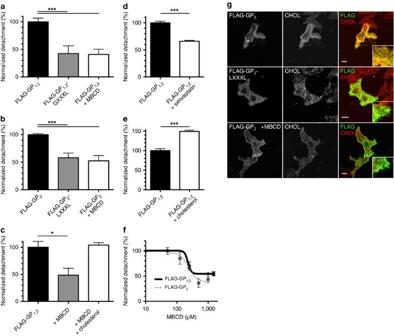Figure 3: MBCD suppresses the detachment of cells induced by Ebola GP. (a,b) HeLa cells were transfected with either FLAG-GP1,2, its mutant FLAG-GP1,2-GXXXL, FLAG-GP2or FLAG-GP2-LXXXL for 24 h. Six hours post transfection, 0.5 mM MBCD was added. The ratio of adherent to detached cells was determined by flow cytometry. (c) The inhibitory effect of MBCD on GP-induced detachment is overcome by the addition of exogenous cholesterol. Cells transfected with FLAG-GP1,2were treated with 5 mM MBCD for 30 min before transfection. Cholesterol was replenished by incubation with 100 μM MBCD-complexed cholesterol for 30 min. (d) Detachment is reduced in statin-treated cells. Cells were cultured in 2 μM simvastatin for 4 days. Cells transfected with FLAG-GP1,2are compared with cells without statin treatment. (e) Exogenous cholesterol increases GP-induced detachment. Cells transfected with FLAG-GP1,2were treated 6 h post transfection with 100 μM MBCD-complexed cholesterol for 30 min. Data points represent the mean±s.d. from three independent experiments (N=3). Detachment of ASGR1-transfected cells was subtracted as unspecific detachment. The results of unpaired, two-tailedt-tests are given. *P<0.05; **P<0.01; ***P<0.001. (f) Titration of MBCD to GP-expressing cells. Cells were transfected with GP1,2or GP2and exposed to different concentrations of MBCD as indicated. The data points represent the mean of three independent experiments (N=3). Error bars represent the s.e.. Best-fit values for a sigmoidal dose response of GP1,2(black solid line) and GP2(dashed grey line) are given. The IC50of MBCD-mediated inhibition of detachment by GP1,2was 197.5 μM±25.44 s.e., and 295.1 μM±98.52 s.e. for GP2. (g) Cholesterol enriches in GP2-induced plasma membrane protrusions. HeLa cells were transfected with FLAG-GP2or FLAG-GP2-LXXXL, and treated with 0.5 mM MBCD 6 h post transfection. Cells were fixed and stained with filipin (cholesterol) and anti-FLAG antibodies. Green, FLAG-GP2/FLAG-GP2-LXXXL; red, cholesterol. Scale bar, 20 μm. Figure 3: MBCD suppresses the detachment of cells induced by Ebola GP. ( a , b ) HeLa cells were transfected with either FLAG-GP 1,2 , its mutant FLAG-GP 1,2 -GXXXL, FLAG-GP 2 or FLAG-GP 2 -LXXXL for 24 h. Six hours post transfection, 0.5 mM MBCD was added. The ratio of adherent to detached cells was determined by flow cytometry. ( c ) The inhibitory effect of MBCD on GP-induced detachment is overcome by the addition of exogenous cholesterol. Cells transfected with FLAG-GP 1,2 were treated with 5 mM MBCD for 30 min before transfection. Cholesterol was replenished by incubation with 100 μM MBCD-complexed cholesterol for 30 min. ( d ) Detachment is reduced in statin-treated cells. Cells were cultured in 2 μM simvastatin for 4 days. Cells transfected with FLAG-GP 1,2 are compared with cells without statin treatment. ( e ) Exogenous cholesterol increases GP-induced detachment. Cells transfected with FLAG-GP 1,2 were treated 6 h post transfection with 100 μM MBCD-complexed cholesterol for 30 min. Data points represent the mean±s.d. from three independent experiments ( N =3). Detachment of ASGR1-transfected cells was subtracted as unspecific detachment. The results of unpaired, two-tailed t -tests are given. * P <0.05; ** P <0.01; *** P <0.001. ( f ) Titration of MBCD to GP-expressing cells. Cells were transfected with GP 1,2 or GP 2 and exposed to different concentrations of MBCD as indicated. The data points represent the mean of three independent experiments ( N =3). Error bars represent the s.e.. Best-fit values for a sigmoidal dose response of GP 1,2 (black solid line) and GP 2 (dashed grey line) are given. The IC 50 of MBCD-mediated inhibition of detachment by GP 1,2 was 197.5 μM±25.44 s.e., and 295.1 μM±98.52 s.e. for GP 2 . ( g ) Cholesterol enriches in GP 2 -induced plasma membrane protrusions. HeLa cells were transfected with FLAG-GP 2 or FLAG-GP 2 -LXXXL, and treated with 0.5 mM MBCD 6 h post transfection. Cells were fixed and stained with filipin (cholesterol) and anti-FLAG antibodies. Green, FLAG-GP 2 /FLAG-GP 2 -LXXXL; red, cholesterol. Scale bar, 20 μm. Full size image On the basis of the immunofluorescence analysis of cells expressing FLAG-GP 2 and co-stained for actin, we observed microfilaments at the basis of the FLAG-GP 2 -induced filaments ( Fig. 1b and Fig. 2a,b ). We therefore incubated the cells with cytochalasin B (CB), an inhibitor of actin filament polymerization, and observed that GP 2 -transfected cells no longer exhibited GP-induced filaments, although FLAG-GP 2 was significantly localized to the plasma membrane ( Supplementary Fig. 3d ), which suggested a role for actin in the observed phenotype, that is, potentially acting as a scaffold for GP-induced filaments. Cholesterol impacts GP-induced cytotoxicity Notably, the endomembrane system in FLAG-GP 1,2 - and FLAG-GP 2 -transfected cells appears unaffected ( Supplementary Fig. 2a,b ). The partitioning of GP into (cholesterol-dependent) detergent-resistant membranes [40] suggested that in addition to the GXXXA motif, the oligomerization of GP might be affected through the increased level of cholesterol at the plasma membrane. A cholesterol gradient exists across the secretory pathway [41] (low in the endoplasmic reticulum (ER) and high in the plasma membrane), and would hence allow the formation of filaments at the plasma membrane, but not in the endomembrane system. To analyse the specific interactions of GP with cholesterol, we utilized a well-established photoaffinity-labelling assay [42] , [43] , [44] , [45] . Radioactively labelled (tritiated) photoactivatable cholesterol was fed to HeLa cells expressing either FLAG-GP 1,2 , FLAG-GP 2 or their respective variants. At 24 h post transfection, the cells were irradiated with ultraviolet, thereby crosslinking the photolabile cholesterol analogue to the proteins and lipids in the immediate proximity (≤3 Å). As a control, the equally trimeric and plasma membrane-resident protein ASGR1 was employed. Although ASGR1 exhibited weak labelling despite high expression levels ( Supplementary Fig. 3e ), both FLAG-GP 1,2 and FLAG-GP 2 were highly and efficiently labelled ( Fig. 2e ). SDS-resistant oligomers of FLAG-GP 2 corresponding to dimers and trimers were observed. Strikingly, a strong reduction in photocholesterol labelling was observed for both FLAG-GP 1,2 -GXXXL and FLAG-GP 2 -LXXXL ( Fig. 2e ). The reduction in cholesterol labelling of the GXXXA motif point mutants was correlated with a strong decrease in cell detachment of ∼ 50%, respectively ( Fig. 3a,b ). Therefore, we next analysed the effect of lowering cholesterol in the plasma membrane of FLAG-GP 2 and FLAG-GP 1,2 -transfected cells with regard to filament production and cell detachment. Methyl-β-cyclodextrin (MBCD) is a well-established tool for lowering the cholesterol content in the plasma membranes of mammalian cells [46] . We exposed cells transfected with full-length FLAG-GP 1,2 , FLAG-GP 2 or variants mutated in the central GXXXA motif to 0.5 mM MBCD at 6 h post transfection, which significantly lowered the levels of cholesterol at the time of analysis 24 h post transfection (>25%; Supplementary Fig. 4a ). Subsequently, we measured the extent of detachment induced through the respective proteins in the presence and absence of MBCD using flow cytometry and immunofluorescence. Strikingly, MBCD significantly reduced (>50%) the level of detachment induced through FLAG-GP 1,2 and FLAG-GP 2 constructs ( Fig. 3a,b ), whereas for FLAG-GP 1,2 -GXXXL and FLAG-GP 2 -LXXXL, detachment was not affected after treatment with MBCD ( Supplementary Fig. 3b ). Treatment with MBCD alone did not significantly induce the detachment of cells, changes in morphology or interfered with expression of GP ( Supplementary Figs 3c, 4c and 7 ). Accordingly, when we incubated the cells with the statin simvastatin before transfection, a significant reduction in the cholesterol levels was observed (>30%; Supplementary Fig. 4b ), and GP-induced detachment was significantly reduced ∼ 40% ( Fig. 3d ). Interestingly, the addition of cholesterol to cells using cholesterol-loaded MBCD strongly increased GP-induced cell detachment ( Fig. 3e ). Furthermore, the inhibitory effect of MBCD on GP-induced detachment was restored when the cells were incubated with MBCD-complexed cholesterol ( Fig. 3c ). Next we expanded the analysis of filoviral GP 2 subunits to Marburg virus (MARV) and Lloviu cuevavirus (LLOV), the only two remaining genera of Filoviridae [47] , [48] . Comparisons of the TMDs of the respective GP 2 subunits of these viruses ( Supplementary Fig. 5a ) revealed that EBOV and LLOV share a high extent of sequence identity, including the G/A/S-XXX-G/A/S motif, but that MARV lacks a comparable sequence ( Supplementary Fig. 5b ). Analogous to EBOV GP 2 , we examined FLAG-LLOV- and FLAG-MARV- GP 2 for the induction of cell detachment and production of plasma membrane protrusions. MARV FLAG-GP 2 induced neither virus-like-filament formation at the plasma membrane, nor significant cell detachment, while the GXXXA motif containing LLOV FLAG-GP 2 triggered cell protrusions and cell detachment comparable to EBOV FLAG-GP 2 , and this effect was susceptible to treatment with MBCD ( Supplementary Fig. 5c,d ). These data highlight the correlation between the presence of G/A/S-XXX-G/A/S motifs in the TMD of filoviral GP, cell detachment and cholesterol. Next we employed the cholesterol-specific probe filipin to examine the enrichment of cholesterol in GP 2 -induced cell protrusions [49] . Although GP 2 -expressing cells are efficiently labelled at the plasma membrane and its filamentous protrusions, staining of the plasma membrane is strongly reduced in MBCD-treated cells (concomitant with the absence of protrusions), and FLAG-GP 2 -LXXXL-expressing cells exhibit low filipin co-staining ( Fig. 3g ). We speculate that the co-aggregation of cholesterol into Ebola virions and the concomitant depletion of plasma membrane cholesterol might also contribute to pathogenicity, as the sequestration of cholesterol would also likely affect the function of cholesterol-interacting receptors and signalling proteins in the plasma membrane, such as the T-cell receptor or MHC class II molecules [50] , [51] . Altogether, these data suggest that the GXXXA motif mediates interactions among GP trimers, generating higher, cholesterol-competent, GP oligomers. Thus, the mutation of this motif correlates with a loss of MBCD sensitivity and a marked reduction in detachment. The titration of MBCD revealed a sigmoidal dose response for both GP 1,2 and GP 2 constructs, with half-maximal inhibition of detachment at similar concentrations (FLAG-GP 1,2 : 197.5 μM±25.4 s.e., and FLAG-GP 2 : 295.1 μM±98.5 s.e. ; Fig. 3f ). Thus, we concluded that the cytotoxicity conferred through GP depends on cholesterol and is additionally influenced by the presence of a GXXXA motif in the TMD. Although these data strongly implicated cholesterol as the major lipid involved in cytotoxicity, we cannot exclude that other lipids were indirectly affected in these experiments. A reduction in the cholesterol levels at the plasma membrane might reflect differences in the composition of specific lipid microdomains targeted through GP, for example, polyunsaturated phospholipids resulted in deformations of the plasma membrane [52] , and phosphatidylserine levels in the cytoplasmic leaflet might also be affected. Nonetheless, these data suggest that cholesterol-reducing treatments are potential candidates for therapeutics to counteract the pathogenicity induced through Ebola GP; these treatments could also be employed after infection with Ebola virus as an addition to the established post exposure regimens [53] , [54] , [55] , [56] , [57] , [58] , [59] , [60] . Cyclodextrins have been patented as antiviral agents for the treatment of infections resulting from various enveloped viruses [61] . Treatment with MBCD is even more promising because the IC 50 reported here is ∼ 20-fold lower than those determined for the herpes, vaccinia, Epstein–Barr and hepatitis C viruses [61] . FLAG-GP 2 -induced filaments form by retraction We next monitored the production of the FLAG-GP 2 -induced filaments through live-cell imaging using a TIRF-DIC (total internal reflection fluorescence-differential interference contrast) microscope set-up. As depicted in Fig. 4c and in Supplementary Movie 1 , after 370 min and within the course of ∼ 70 min, the cells contract with filamentous structures left behind while the cell body retracts, which suggests that the filaments are formed through retraction rather than outgrowth. Moreover, bubbles were observed underneath the cell, and the cells rounded up before eventual detachment, which suggests a correlation between the production of plasma membrane protrusions and cell detachment. 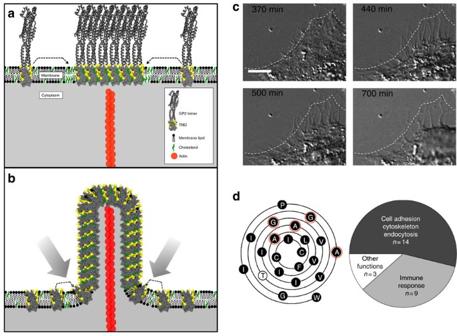Figure 4: A novel role for GP in virus assembly at the plasma membrane. (a) Model depicting the proposed initial steps in the formation of GP2-based domains at the plasma membrane. GP2trimers begin to associate due to elevated levels of cholesterol at the plasma membrane. Interactions among trimers are stabilized via seam-like arranged Gly and Ala residues present in each TMD (highlighted yellow). Black, membrane lipid; green, cholesterol; red, actin; grey/yellow, trimeric TMD of Ebola GP. The TMD was simulated as a solvent-excluded structure using BallView 1.3 and is depicted in grey. The seam-like assembly of glycine and alanine residues is depicted in yellow. Palmitates covalently attached to cysteines 221 and 223 are depicted in blue. The trimeric ectodomain of GP2(PDB ID: 1EBO) is depicted as grey ribbons. Dashed arrows indicate the addition of GP2trimers to a growing cholesterol-dependent aggregate. (b) The cholesterol-dependent GP2-aggregate reaches a critical mass, and collapses around actin filaments in vicinity to the plasma membrane. Dashed arrows indicate the continuous addition of GP2trimers to the aggregate, thereby forcing a contraction around the actin-stabilized nascent filament (indicated by bold grey arrows). Here the trimeric ectodomain of GP2was omitted for clarity. (c) Live-cell differential interference contrast imaging of HeLa cells transfected with FLAG-GP2. Cells were imaged for 16 h at 10 min intervals, 5 h post transfection. Dashed line indicates the territory of the cell before the emergence of filament-like structures. Scale bar, 10 μm. (d) A subset of host membrane proteins exhibit a GP-like TMD architecture. Left, helical wheel representation (Wenxiang diagram67) of the TMD of ZEBOV GP. Polar residues are depicted as white circles, hydrophobic residues in black. Gly and Ala residues contributing to the seam-like assembly are depicted as black circles with red outlines. Right, mammalian single-spanning membrane proteins that contain ≥5 small side-chained residues (Gly, Ala, Ser) in a 180° angle, as observed within the TMD of GP. The pie chart depicts the distribution of the annotated functions of the candidates. Candidates with a role in cell adhesion and organization of the cytoskeleton are depicted in dark grey (n=14); light grey, candidates involved in immune response (n=9); white, candidates with other functions (n=3). Figure 4: A novel role for GP in virus assembly at the plasma membrane. ( a ) Model depicting the proposed initial steps in the formation of GP 2 -based domains at the plasma membrane. GP 2 trimers begin to associate due to elevated levels of cholesterol at the plasma membrane. Interactions among trimers are stabilized via seam-like arranged Gly and Ala residues present in each TMD (highlighted yellow). Black, membrane lipid; green, cholesterol; red, actin; grey/yellow, trimeric TMD of Ebola GP. The TMD was simulated as a solvent-excluded structure using BallView 1.3 and is depicted in grey. The seam-like assembly of glycine and alanine residues is depicted in yellow. Palmitates covalently attached to cysteines 221 and 223 are depicted in blue. The trimeric ectodomain of GP 2 (PDB ID: 1EBO) is depicted as grey ribbons. Dashed arrows indicate the addition of GP 2 trimers to a growing cholesterol-dependent aggregate. ( b ) The cholesterol-dependent GP 2 -aggregate reaches a critical mass, and collapses around actin filaments in vicinity to the plasma membrane. Dashed arrows indicate the continuous addition of GP 2 trimers to the aggregate, thereby forcing a contraction around the actin-stabilized nascent filament (indicated by bold grey arrows). Here the trimeric ectodomain of GP 2 was omitted for clarity. ( c ) Live-cell differential interference contrast imaging of HeLa cells transfected with FLAG-GP 2 . Cells were imaged for 16 h at 10 min intervals, 5 h post transfection. Dashed line indicates the territory of the cell before the emergence of filament-like structures. Scale bar, 10 μm. ( d ) A subset of host membrane proteins exhibit a GP-like TMD architecture. Left, helical wheel representation (Wenxiang diagram [67] ) of the TMD of ZEBOV GP. Polar residues are depicted as white circles, hydrophobic residues in black. Gly and Ala residues contributing to the seam-like assembly are depicted as black circles with red outlines. Right, mammalian single-spanning membrane proteins that contain ≥5 small side-chained residues (Gly, Ala, Ser) in a 180° angle, as observed within the TMD of GP. The pie chart depicts the distribution of the annotated functions of the candidates. Candidates with a role in cell adhesion and organization of the cytoskeleton are depicted in dark grey ( n =14); light grey, candidates involved in immune response ( n =9); white, candidates with other functions ( n =3). Full size image A subset of host proteins exhibits a GP-like TMD arrangement Subsequently, we analysed the amino-acid sequences of host single-spanning plasma membrane-resident proteins to characterize the seam-like arrangement of Gly and Ala residues present in the TMD of GP. Strikingly, only 26 proteins exhibited more than five Gly, Ala or Ser residues within a seam-like arrangement in the TMD. A total of 14 of these candidates were implicated in cell adhesion or cytoskeleton organization ( Fig. 4d , Supplementary Table 1 ). Among these TMDs are known interactors of GP, such as β1-integrin [24] . Nine proteins involved in the immune response (for example, the α-chain of HLA class II) were also identified. These findings suggest that GP 1,2 might bind to and interfere with these candidates via the GXXXA motif. As depicted in Fig. 4a , we propose the following model for the formation of GP-induced filaments—at the onset of assembly, GP-TMDs trimerize in a cholesterol-independent manner. During Ebola virus assembly, trimeric GP subunits interact within cholesterol-enriched membrane domains via GXXXA-motifs in the TMDs, generating a lattice-like structure that predominantly contains GP and excludes host proteins ( Fig. 4a , centre). When a critical lattice size is formed, this membrane domain collapses around an actin filament that serves as a scaffold for plasma membrane filament formation ( Fig. 4b ). Matrix protein VP40 participates in this process through oligomerization at the cytoplasmic face of the plasma membrane [34] , [62] ( Supplementary Fig. 6 ), further stabilizing the filamentous structures in the viral context and putatively additionally exerting an outward-directed force on the plasma membrane. In summary, based on the results obtained in the present study, we propose a novel mechanism for Ebola virus assembly at the plasma membrane, based on cholesterol-dependent interactions among GPs, leading to the collapse of large GP aggregates around actin filaments. Rather than through outgrowth, the formation of these filaments reflects the growth of GP aggregates within the plasma membrane and the subsequent wrapping of these aggregates around actin scaffolds ( Fig. 4a,b ). This mechanism might be closely associated with cell detachment, and suggests two novel drug targets to counter GP-mediated cell detachment—cholesterol, which could be targeted using cholesterol-reducing agents, such as MBCD and statins, and the central GXXXA-motif situated within a seam-like assembly of Gly and Ala residues in the TMD of GP. Reagents and antibodies MBCD, simvastatin, CB, water-soluble cholesterol, phalloidin-conjugated to Atto 565, Filipin III and EZview red anti-FLAG M2 affinity gel were purchased from Sigma-Aldrich. Prolong Gold Antifade reagent containing 4′,6-diamidino-2-phenylindole, 5-hexadecanoylaminofluorescein and WGA conjugated with Alexa 647 were purchased from Life Technologies. Cell dissociation buffer was purchased from Gibco. The following antibodies were purchased from Life Technologies—Alexa Fluor 546 goat anti-mouse, Alexa Fluor 546 goat anti-rabbit, Alexa Fluor 546 donkey anti-sheep, Alexa Fluor 488 goat anti-rabbit, Alexa Fluor 488 goat anti-mouse. Anti-FLAG mouse and anti-FLAG rabbit were purchased from Sigma. Anti-GM130 mouse was purchased from BD-Transduction, anti-TGN46 sheep was obtained from Serotec and anti-Calnexin rabbit from Abcam. Plasmids and constructs FLAG-tagged cDNA for Ebola GP 2 and GP were purchased as synthetic genes from GeneArt (Life Technologies) based on the reverse-translated amino-acid sequences of Uniprot Q05320 (VGP_EBOZM) using the most likely codon usage for H. sapiens ( Supplementary Table 2 ). Using EcoRI and NotI sites, the synthetic genes were cloned into pEGFP-N1 vectors, from which EGFP had been removed via EcoRI/NotI digestion. Site-directed mutagenesis was performed using the QuikChange Site-Directed Mutagenesis Kit (Stratagene). FLAG-tagged ASGR1-cDNA was obtained from Origene (clone # RC205686). Cell culture and transfection HeLa cells (DSMZ number: ACC 57) were cultured in α-MEM (Applichem) with 10% fetal calf serum (FCS), 2 mM L -glutamine and 100 U ml −1 penicillin, 100 μg ml −1 streptomycin. HEK 293 T (DSMZ number: ACC 305), COS-7 (DSMZ number: ACC 305) and Vero (ECACC 84113001) cells were cultured in DMEM (Applichem) supplemented with 10% FCS, 4 mM L -glutamine and 100 U ml −1 penicillin and 100 μg ml −1 streptomycin at 5% CO 2 and 37 °C. Transfection was performed using FuGENE HD transfection reagent (Promega) according to the manufacturer’s instructions (3 μg DNA per 9 μl FuGENE HD per well of a six-well plate). HUVEC cell culture and transfection Human umbilical vein endothelial cells (HUVECs) from single donors (PromoCell) were cultured in Endopan 3 Kit medium (PAN-Biotech) supplemented with 10% fetal bovine serum, 100 U ml −1 penicillin and 100 μg ml −1 streptomycin (Gibco Life Technologies) in a 5% CO 2 humidified incubator at 37 °C. HUVECs were used between passage 1 and 5. For microscopy studies, HUVECs were plated onto glass coverslips coated with 0.1% gelatin (from porcine skin; Sigma-Aldrich). For transfection, the culture medium was removed from a monolayer of 90% confluent cells. The cells were washed with PBS (1 × ; PBS, Sigma-Aldrich) and subsequently trypsinized (0.05% Trypsin-EDTA; Gibco by Life Technologies). A total of 1.5 × 10 6 cells were resuspended in a final volume of 400 μl of electroporation buffer (RPMI-1640-medium supplemented with 10% fetal bovine serum) and placed in a 0.4 cm electrode gap cuvette (PEQLAB). 15 μg FLAG-GP 2 was mixed with the cell suspension and incubated at 4 °C for 10 min. Cells were electroporated using an electric pulse generator (BioRad Gene Pulser Xcell) under the following conditions—square wave electric pulse, 250 V and 40 ms pulse length. Subsequently, the cells were resuspended in the respective growth media and plated for further assays. After 4 h, the culture medium was replaced with fresh complete growth medium. The images were acquired after 24 h through confocal microscopy using a Zeiss LSM 510 unit mounted on an Axiovert 200 inverted microscope with a 1.4 Plan-APOCHROMAT × 63 oil objective. Confocal microscopy The cells were plated on 35 mm glass-bottomed dishes (MatTek Corp.) and transfected using FuGENE HD. After 24 h, the cells were washed three times with PBS (pH 7.4) and fixed with 3.6% paraformaldehyde (Sigma-Aldrich) for 20 min on ice. For endomembrane staining, the cells were permeabilized using 0.5% (w/v) Triton-X-100 for 5 min at RT. After washing three times, for blocking, cells were incubated with 1% bovine serum albumin (BSA; Carl Roth) in PBS for 1 h. Immunofluorescence was performed with a dilution of primary antibodies at 1:200 and secondary antibodies at 1:1,000 in 0.5% BSA in PBS. The primary antibody dilutions were added to the cells for 1 h, followed by washing three times with PBS for 5 min. Secondary antibody dilutions were subsequently added for 30 min. Alexa647-conjugated WGA was used at final concentration of 10 μg ml −1 for 20 min, and 10 nmol of Atto565-conjugated phalloidin (Sigma) was added to 1 ml of methanol and incubated with the cells at a dilution of 1:100 in PBS for 30 min. The samples were examined through confocal microscopy using a Zeiss LSM 510 unit mounted on an Axiovert 200 inverted microscope with a 1.3 NA Plan-NEOFLUAR × 40 oil objective, equipped with an argon laser. Image processing was performed using Zen 2011 and ImageJ software. Quantification of cell detachment using flow cytometry The cells were plated on 6-well dishes (Corning Inc.) and transfected with the indicated contructs using FuGENE HD. At the indicated timepoints, the dishes were placed on ice. The culture medium containing detached cells was transferred to 1.5 ml tubes and centrifuged for 6 min (10,000 r.p.m.). The supernatant was discarded, and the pellet was resuspended in 200 μl serum-free DMEM. The adherent cells were washed once with PBS, and subsequently incubated with 300 μl of EDTA-containing cell dissociation buffer (Gibco) at 37 °C for 5 min. Subsequently, 300 μl of serum-free DMEM was added and the resuspended cells were transfered to 1.5 ml tubes. The ratio of detached versus total cells was quantified using a FACSCalibur flow cytometer (Beckton Dickinson). Fluorescence stain of membrane cholesterol and quantification A filipin stock solution was prepared in dimethylsulphoxide at a concentration of 50 mg ml −1 . For membrane staining, unpermeabilized paraformaldehyde-fixed cells were incubated with a 1:100 dilution of filipin solution in PBS containing 1% BSA for 30 min before incubation with the antibodies (primary antibody: 1:200; secondary antibody: 1:1,000) and then subjected to confocal microscopy. To quantify the membrane cholesterol population, six-well plates with adherent cells were treated accordingly, and filipin fluorescence was measured using a MolecularDevices SpectraMax M5 microplate reader at an excitation wavelength of 355 nm and emission wavelength of 460 nm (ref. 49 ). Treatment of cells with MBCD and CB A stock solution of CB was prepared at 5 mg ml −1 in dimethylsulfoxide. To deplete cholesterol and inhibit actin polymerization, MBCD and CB were added to the medium at the concentrations indicated 6 h post transfection and incubated overnight. Bioinformatics All proteins annotated as membrane proteins were downloaded from Uniprot [63] . These proteins were homology reduced to 30% using CD-HIT [64] . To map the TMDs of these proteins, we used DG-pred [65] with the constraint that a TMD shows a Δ-G score <0. To identify putative TMD–TMD interaction interfaces that were enriched in the Gly, Ala and Ser residues, we generated an algorithm that analyses the TMDs from the z axis. On the basis of the assumption of the regular spacing of the residues in these alpha-helical segments, the total number of small side chain-containing residues (Gly, Ala and Ser) and the relative distribution of these residues around the TMD were obtained. Three data sets corresponding to the different subcellular localizations of the membrane proteins (ER, Golgi and plasma membrane) were generated. To evaluate the data, the plasma membrane protein data set was analysed for proteins containing ≥5 residues of Gly, Ala or Ser positioned at an angle of 180°—as observed in the TMD of Ebola GP ( Fig. 4d ). Falsely annotated entries and those specific to early developmental stages and proteins exclusively present in certain tissues were omitted for clarity. Depletion and replenishment of cholesterol in the cells MBCD-complexed cholesterol from Sigma was added to the cells at 6 h after transfection for 30 min at a concentration of 100 μM in normal growth medium. The cells were washed with PBS and incubated overnight in growth medium. For the rescue experiments, the cells were incubated in 5 mM MBCD for 60 min before transfection and washed three times with PBS. At 6 h after transfection, water-soluble cholesterol was added as indicated. Treatment of cells with a statin The cells were cultured in simvastatin at 2 μM for 4 days before experiments in normal growth medium. The cells then were subsequently transfected and treated as described above. Scanning electron microscopy The cells were plated onto 35 mm glass-bottomed dishes (MatTek), and transfected for 24 h with different GP variants. The cells were fixed with 2% glutaraldehyde in 0.1 M sodium phosphate buffer (Sørensen), pH 7.4 for 2 h, rinsed with buffer and dehydrated with an ascending series of ethanol. The samples were critical point dried using carbon dioxide and the slides were coated with gold (5 nm). The samples were analysed using a ZEISS ULTRA 55-field emission scanning electron microscope, using the Everhart–Thornley secondary electron detector. Live-cell imaging HeLa cells were plated onto 35-mm MatTek glass-bottomed dishes and transfected for 24 h with 3.3 μg FLAG-GP 2 and 10 μl FuGENE HD transfection reagent in complete DMEM medium. After 5 h, the cells were washed with PBS and a HEPES-based imaging medium (Invitrogen). Microscopy was performed on a Nikon TIRF-2 system with Eclipse Ti inverted microscope, using a Nikon Apo-TIRF 1.5 NA × 60 oil objective in differential interference contrast mode with a Hamamatsu 1394 ORCA-ERA camera and an incubation chamber adjusted to 37 °C and 5% CO 2 . Imaging was commenced at 5 h post transfection, with an acquisition rate of one image per 10 min, for a total duration of 16 h using NIS-Elements Microscope Imaging Software. In vivo photoaffinity labelling with cholesterol FLAG-tagged GP 2 and GP 1,2 constructs and variants thereof and ASGR1, as a negative control, were probed for protein–cholesterol interaction in vivo . For this purpose, photoactivatable cholesterol was employed for photolabelling experiments as previously described [66] . In brief, HeLa cells were grown in six-well dishes and transfected using FuGENE HD (1 μg DNA+3 μl transfection reagent in 100 μl Opti-MEM (Invitrogen) at ∼ 60% confluency. After 16 h, the cells were labelled with 75 μCi of ( 3 H)-photocholesterol in 3 ml of DMEM supplemented with 10% delipidated FCS for 8 h. The cells were ultraviolet irradiated for 10 min on ice and lysed for 1 h in 100 μl lysis buffer (50 mM HEPES-NaOH, pH 7.4, 100 mM NaCl, 5 mM EDTA, 1% Triton-X-100 (v/v), 0.5% deoxycholate (w/v), and protease inhibitor cocktail (cOmplete mini, Roche)). Post-nuclear supernatants were subjected to immunoprecipitation using M2-(anti-FLAG)-affinity gel (Sigma-Aldrich) according to the manufacturer’s instructions. The proteins were subsequently eluted in 4 × SDS–polyacrylamide gel electrophoresis sample buffer containing 16% SDS and subjected to SDS–polyacrylamide gel electrophoresis (10–20% Tris/Tricine gradient gels, Invitrogen), western blotting and the quantitative immunodetection of FLAG-tagged proteins using a LI-COR infrared imager. Radioactively labelled proteins were detected by digital autoradiography (Beta Imager 2000, Biospace Lab), using acquisition times of 16 h. How to cite this article: Hacke, M. et al. Inhibition of Ebola virus glycoprotein-mediated cytotoxicity by targeting its transmembrane domain and cholesterol. Nat. Commun. 6:7688 doi: 10.1038/ncomms8688 (2015).